Bird–flower visitation networks in the Galápagos unveil a widespread interaction release Owing to food scarcity and to the high densities that vertebrates often reach on islands, typical insect- and seed-eaters widen their feeding niche and interact with a greater fraction of species than their mainland counterparts. This phenomenon, coined here ‘interaction release’, has been previously reported for single species but never for an entire community. During 4 years, we gathered data on bird–flower visitation on 12 Galápagos islands. We show that all sampled land birds exploit floral resources and act as potential pollinators across the entire archipelago, in all major habitats and all year round. Although species and link composition varies among islands, strong interaction release takes place on all islands, making their bird–flower network highly generalized. Interaction release is crucial to the survival of native birds but simultaneously threatens the unique biodiversity of this archipelago, as the birds also visit invading plants, likely facilitating their integration into pristine native communities. ‘I took great pains in collecting the insects, but excepting Tierra del Fuego, I never saw in this respect so poor a country ’, goes the famous Darwin quote [1] about the insect fauna on the Galápagos. These islands, as well as other isolated oceanic islands, typically sustain a low diversity of, not just insects, but plants and animals in general, and thus have a more simple interaction structure compared with mainland biota [2] , [3] , [4] , [5] . Consequently, island species experience a release in their interaction structure, promoting the exploitation of new interaction possibilities. Indeed, islands have a high proportion of generalist species showing novel and opportunistic interactions [2] , [6] , [7] . We term this niche expansion process ‘interaction release’ (as one aspect of the wider concept ‘ecological release’ [8] ), that is, island species wire up novel mutualists and prey as a response to mutualist and food shortage, and to reduced predation risk. To study the generality of this phenomenon at the community level, we adopted a network approach [9] , [10] , [11] . Single species of insect-eating birds and lizards are known to supplement an insect-poor diet with nectar, pollen and fruit [12] , [13] , [14] , [15] . Such interaction release is common, especially among density-compensators, that is, species that respond to low interspecific competition and reduced levels of predation and parasitism in their habitat by increasing their population size. Density-compensating vertebrates often behave as super-generalists and may exert strong directional selection on their interacting partners [16] , [17] , [18] . In particular, super-generalist vertebrates may be important to plants suffering from reduced reproductive output due to a scarcity of insect pollinators. Empirical support for such a scenario is still scant but growing [19] , [20] . For most of the Galápagos land bird fauna (19 out of 23 species), we evaluated the extent of its interaction release towards the use of floral resources such as nectar and pollen. These birds are generally regarded as insect- and seed-eaters [21] , but a shortage of these resources, at least of insects, may force birds to expand their food niche to include floral rewards, abundant and widespread across all islands. We estimated pollen harvesting through direct observation of flower visits and inspection of pollen load on birds’ beak and plumage. A recent literature review reported only a total of 20 interactions between Galápagos birds and flowering plants [22] , and at least one of them demonstrated effective pollination [14] . However, no study has screened any island bird fauna in the world for its potential importance as pollinators. In this respect, the most detailed available information is about flowers visited by New Zealand birds [23] . First, we built a qualitative archipelago-wide bird–flower interaction network based on data from 12 Galápagos islands to assess bird pollination patterns across the archipelago. In addition, based on a full year of pollination surveys in the two main habitats on two more intensively studied islands (Santa Cruz and San Cristóbal), we constructed one quantitative network per island, per habitat (lowland and highland) and per season (hot and cold). The strength of an interaction between plant species i and bird species j was scored as the frequency of occurrence of pollen from i in samples from j . Network structure was evaluated by a set of network descriptors. Note that, throughout the manuscript, we refer to birds as pollinators regardless of their effectiveness. The land bird community on the Galápagos shows strong interaction release by exploiting floral resources and thus acting as potential pollinators across the entire archipelago. Birds—including virtually all finches, the yellow warbler and the Galápagos flycatcher—visit flowers extensively throughout the year, and both in the arid and humid zone, and a high spatio-temporal structural network consistency is found. At present, we expect it to be a general oceanic island phenomenon, but no comparable data are yet available. This behavioural response across the whole bird community may be crucial to the survival of both native birds and plants, but unfortunately also catalyses the integration of invading plants into the natural systems of these unique islands. Archipelago-wide patterns All of the 19 bird species examined (representing 83% of Galápagos native land birds) were found to feed on flowers and/or transport pollen of 106 plant species ( Fig. 1 ). 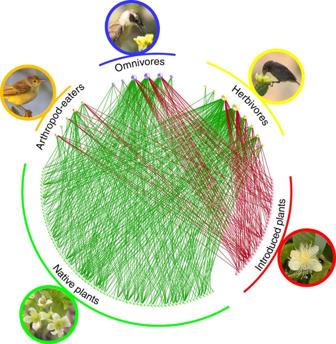Figure 1: Archipelago network in which all interactions observed on the 12 largest Galápagos islands were pooled. This network consisted of 19 land bird species (all but 2 being endemic to the islands) and 106 plant species, either native (green nodes) or introduced (red nodes) to the islands. Birds were classified into three functional groups depending on their main diet composition. Note that granivores, nectarivores and folivores (three groups frequently overlapping) are merged into the herbivore category. Most birds were highly generalized (their generalization level is proportional to node size), each pollinating an average of 22 plant species (range 1–77). Total number of network links was 421 (increasing 20 times the previously known number of flower–bird interactions in the archipelago). Among the main bird hubs were two finch species, the yellow warbler and the Galápagos flycatcher. Nearly a third of all identified plant species were introduced. Such species are all endemic to Galápagos, except the native Coccyzus melacoryphus and Dendroica ( Setophaga) petechia ( Supplementary Table 1 ). Thus, irrespective of the main feeding guild of these 19 bird species, the whole bird community expanded its niche and included floral rewards into the diet. The other four land bird species could not be included in this study because they are either very rare or absent in the study areas ( Supplementary Table 1 ). We know, however, that at least two of those four species, the criticaly endangered Camarhynchus pauper and Mimus trifasciatus from Floreana Island, do visit flowers ( Supplementary Table 1 ). One hundred out of the 106 plant species were identified to species or genus level; 55 were trees or shrubs, 28 were herbs and 17 were vines; ∼ 30% of these plants were endemics, 41% natives and 29% aliens to Galápagos ( Fig. 1 ). 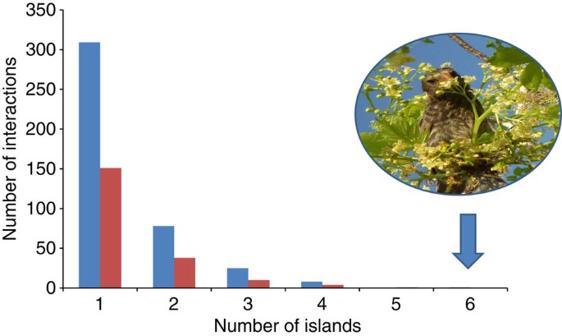Figure 2: Number of plant–bird interactions found on different number of islands. Blue columns correspond to the interactions pooled from all 12 islands (archipelago network), whereas red columns correspond to the 5 islands where our sampling effort was similar (Fernandina, Pinta, Santiago, Santa Cruz and San Cristóbal). Only one interaction—Geospiza fuliginosaandBursera graveolens(photo inset)—was observed on a maximum of six islands. Each island had a high diversity of bird–flower interactions that were ‘single-island endemics’, strongly enhancing the uniqueness of each island. Despite this variation, the observation of ‘interaction release’ was general across the archipelago. Thus, birds visited both native and alien plants ( Supplementary Table 2 ), with only a weak preference for natives (mean±s.d.=4.48±3.53 links to native species ( n =46) and 3.38±3.58 links to alien species ( n =24); GLM: z =2.45, P <0.01). Two of the most visited plants were highly invasive aliens: Psidium guajava and Impatiens balsamina , being visited by 14 and 12 bird species, respectively. The combined archipelago network had a connectance of 21% ( Supplementary Table 2 ). Most bird individuals transported numerous pollen grains (mean±s.d.=233±1,065 pollen grains; median=5; maximum=20,112; n =769 samples). About 65% of all sampled pollen loads were mixed, that is, included pollen from several plant species (mean±s.d.=2.45±1.56 pollen species per sample; median=2; max=10; n =502). Two finches ( Geospiza fuliginosa and G. fortis ), the Galápagos flycatcher ( Myiarchus magnirostris ) and the yellow warbler ( D. petechia ) were the most abundant and generalized, being involved in 54% of all network links, that is, these four bird species showed the strongest interaction release. Almost all species-rich pollination networks are both nested [24] and modular [25] . However, the archipelago network was only nested (NODF=61.80, P <0.001), and not modular ( M =0.27, P >0.05), that is, the whole network operated as one module. Figure 1: Archipelago network in which all interactions observed on the 12 largest Galápagos islands were pooled. This network consisted of 19 land bird species (all but 2 being endemic to the islands) and 106 plant species, either native (green nodes) or introduced (red nodes) to the islands. Birds were classified into three functional groups depending on their main diet composition. Note that granivores, nectarivores and folivores (three groups frequently overlapping) are merged into the herbivore category. Most birds were highly generalized (their generalization level is proportional to node size), each pollinating an average of 22 plant species (range 1–77). Total number of network links was 421 (increasing 20 times the previously known number of flower–bird interactions in the archipelago). Among the main bird hubs were two finch species, the yellow warbler and the Galápagos flycatcher. Nearly a third of all identified plant species were introduced. Full size image Bird–plant interactions differed strongly among islands, that is, inter-island turnover of interactions was high. Of all scored interactions, 73.4% were from one island, whereas only 2% were found on four or more islands ( Fig. 2 ). To assess to what extent such a finding was due to sampling incompleteness (that is, links missing due to insufficient sampling), we obtained rarefaction curves and asymptotic species richness estimators for each bird species (see Methods). We estimated that we had detected a large fraction ( ∼ 70%) of all existing interactions ( Supplementary Fig. 2 , Supplementary Table 3 ); hence, more sampling would certainly have led to more interactions, but also to more plant species being included in the network. The same high turnover of interactions was found when considering only the interactions observed on a standardized 3-day period during the peak of the flowering season (February of 2010 and 2011) on five of the islands in which we invested an equivalent sampling effort. Figure 2: Number of plant–bird interactions found on different number of islands. Blue columns correspond to the interactions pooled from all 12 islands (archipelago network), whereas red columns correspond to the 5 islands where our sampling effort was similar (Fernandina, Pinta, Santiago, Santa Cruz and San Cristóbal). Only one interaction— Geospiza fuliginosa and Bursera graveolens (photo inset)—was observed on a maximum of six islands. Each island had a high diversity of bird–flower interactions that were ‘single-island endemics’, strongly enhancing the uniqueness of each island. Despite this variation, the observation of ‘interaction release’ was general across the archipelago. Full size image Spatio-temporal variation in network parameters Santa Cruz and San Cristóbal showed very similar network structure despite only 21% of all interactions being shared between them (that is, the same species pair interacting on both islands). Both networks had a high connectance (>30%), high interaction evenness, high species strength and low network specialization ( H ′ 2 )— Supplementary Table 4 and Supplementary Fig. 3 . The interaction pattern was also very similar between the two habitats, although lowlands have higher species richness ( Supplementary Table 4 ) and only 31% of the interactions were shared. On both islands and in both habitats, the endemic small ground finch G. fuliginosa and the alien plant P. guajava were the most connected species. Other plants frequently visited by birds were the endemic prickly pear cactus Opuntia echios and the non-endemic native tree Bursera graveolens in the lowland. The lowland and highland networks were, to some extent, coupled; some species of Opuntia , characteristic of the lowlands, were found in the bird samples from the highlands, suggesting that birds make altitudinal movements. Network structure was also similar between seasons, though the number of interactions was almost twice as high in the hot (wet) season, when most plants were in flower, than in the cold (dry) season ( Supplementary Table 4 ). Only 25% of all interactions were present in both seasons. G. fuliginosa was the all-year-round network hub, together with two other finches ( G. fortis and Camarhynchus parvulus ) in the hot season, and the flycatcher M. magnirostris in the cold season. The main plant hubs were P. guajava in the hot season, whereas the native creeper Galactia striata and the alien herb I. balsamina were cold-season hubs. Comparison between alien and native plants Alien and native plants on Santa Cruz and San Cristóbal islands had a similar number of bird flower visitors (GLM: z =0.92, P =0.36; Supplementary Fig. 4 ) and they differed neither in specialization level d′ ( t =0.93, P =0.35) nor in species strength ( t =0.49, P =0.62), indicating that alien species were fully integrated into the networks. Indeed, some of them had even achieved a central position as network hubs: P. guajava got 32% of all links on San Cristóbal and 14% on Santa Cruz ( Supplementary Fig. 4 ). Comparison across bird functional groups Interaction release was observed in all three functional groups, that is, insectivores, herbivores and omnivores ( Supplementary Table 1 ). The number of flowering plants included in their diet (linkage level) showed a higher average for herbivores (mean±s.d. : 30.6±19.6; n =5) than for arthropod-eaters or omnivores (17.8±15.5 and 14.3±11.3, n =5 and n =4, respectively) though differences were not significant (all P values>0.05). Likewise, no differences were found on the specialization level ( d ′) and interaction strength across functional groups ( Supplementary Fig. 5 ). We demonstrate that bird–flower visitation and pollen transport are very common on the Galápagos Islands. Almost all land birds in the archipelago are involved, visiting over a hundred flowering plant species. Such a massive food-niche widening–that is, interaction release—has never been described for any vertebrate community in the world. Given the lack of similarly detailed studies on other parts of the word, it is too early to say if the massive interaction release we observed is unique to Galápagos or if it might be found elsewhere if detailed screening protocols were implemented. Unfortunately, bird pollination is still rarely reported at the community and network level. In a sample of 53 pollination networks, including ∼ 10,000 plant and animal species, only 9 contained birds: a total of 26 species, of which 19 were hummingbirds ( Supplementary Table 5 ). The vast majority of animals in those pollination networks were insects. Thus, based on this set of networks, we have to conclude that bird pollination within a given habitat is either a rare phenomenon globally or systematically under-reported (perhaps exacerbated by human-caused reduction in bird densities). A massive interaction release might well occur in other archipelagos, where other phenomena like lizard pollination are known to be frequent [12] . A lack of comparable data sets from other archipelagos precludes us from making further conclusions. However, we attempted to calculate similar network parameters for New Zealand, which is the archipelago with most studies of bird pollination. The New Zealand data originate from flower observations, and most of these are from specific plants and birds of high conservation priority, whereas our data mostly come from bird–pollen load analysis. Out of 35 New Zealand land bird species for which we obtained published information [23] , 22 (63%) were observed to visit flowers (compared with the 83% we scored in Galápagos). The New Zealand birds visited 73 plant species, yielding a connectance of 12%, which is still considerably lower than the 21% found in the Galápagos network. Taking into account that the Galápagos network has more species than the New Zealand network, this difference in connectance becomes even larger ( Supplementary Fig. 6 ). Without further information we cannot conclude whether this difference is real or methodological. However, one important characteristic of New Zealand bird biota, which should make flower visitation by birds more frequent, is its honeyeater birds, which belong to an old species-rich phylogeny of nectar-drinking and insect-eating birds. In spite of that, we have to conclude that the land birds of New Zealand seem to respond less massively to flowers than the Galápagos bird fauna. The reasons might be that Galápagos is more isolated, less disturbed and very likely poorer in insects than New Zealand. In addition, a review on the presumed diet of all extant and known extinct native birds in New Zealand concluded that there had been no extinctions from the major nectarivore guild [26] . We also explored how the Galápagos bird–flower network differed from other available bird-flower networks. To do so, we compiled 24 hummingbird–flower networks, all from the mainland or continental islands (Trinidad) ( Supplementary Table 6 ). We compared their levels of connectance, nestedness and modularity with similar values from Galápagos and New Zealand. Correcting for variation in species richness, we found that the Galápagos network had a connectance 50% higher than expected ( Supplementary Fig. 6a ), and the standardized level of nestedness ( z -score) for the Galápagos network was 1.9 times as high as expected ( Supplementary Fig. 6b ). A high connectance may have a strong stabilizing role via functional redundancy, and a nested interaction pattern of interactions might also facilitate the maintenance of species coexistence [27] , provide resistance against perturbations [28] and maximize total abundance [29] . However, there is currently a strong debate about the stabilizing role of nestedness [30] . The lack of modules in the Galápagos bird–flower network is attributed to the large bulk of interactions among generalists [25] , [31] , which glues all species tightly together. The hummingbird networks were also non-modular, except for two networks ( Supplementary Fig. 6c–f , Supplementary Table 6 ). Modularity also influences network stability against disturbances [28] , although the precise role of modularity to network stability depends on the type of disturbance and also on the applied measure of stability (for example, species or community persistence). Thus, a low level of modularity might reduce robustness against an invasion of a parasite or an extinction of a highly connected species, but might be more robust against random secondary species extinctions [32] . Bird pollination may be particularly prevalent in Galápagos because birds of the families visiting flowers in the islands were already preadapted to visit flowers in their original mainland populations. We tested this by compiling all known bird–flower interactions involving those five bird families in South America ( Supplementary Data set 1 ). In general, the flower-visiting Galápagos birds belonging to these five families are regarded as arthropod-eaters (for example, Yellow Warbler, the Galápagos Flycatcher) and granivores (for example, ground finches) [21] . Members of these families are also known to visit flowers in South America, but to a much lower extent: mean S. America=16.3% of the species in the family, mean Galápagos=82.1%; GLMM: F 1,4 =8.8, P =0.041; Supplementary Table 7 ). A rare exception is Dacnis cayana (Thraupidae), which feeds frequently on the flowers of many (≥20) plant species. In addition, Galápagos birds visit a much higher number of plant species than their mainland counterparts (S. America=1.7, Galápagos=23.6; F 1,4 =12.1; P =0.025, Supplementary Table 7 ). Our interaction release hypothesis rests on the assumption that the islands are poor in arthropods. Such an assumption has some support [12] , [33] , [34] , but needs validation from Galápagos. The overall insect species richness of the archipelago is well-known, but insect abundance and biomass are unknown [35] . We did find some evidence of insect poverty in an earlier study from Galápagos [11] , where we scored a connectance C =5% between native insect species visiting the flowers of native plant species. This figure is lower than we should expect (8.4), if we use the regression model in ref. 9 ; C =13.83 exp(−0.003 S ), where S is number of plant and animal species). Moreover, we suggest that birds play a relatively large role compared with insects in the pollination networks of the Galápagos. Our support for this is a tentative comparison of the bird–flower network from this study with the insect–flower network also from Galápagos [11] . These two networks have different link currency, that is, the bird–flower links are based on pollen load and/or flower visitation, whereas the insect–flower links only are based on visitation. We pooled the bird–flower and the insect–flower networks into a total pollination network for the archipelago. The total matrix included 125 plant species, 19 bird species and 213 insect species. Birds and insects shared 40 of the 125 plant species. Nineteen plant species had only insect pollinators, and 66 had only bird pollinators. Thus, although birds only constituted 8% of the total pollinator fauna, and only made 36% of all links, they alone interacted with 53% of the flora, and together with insects with an additional 32% of the plants, thus contributing to the pollination of 85% of the flora. In addition, birds had a central position in the total network because they had a significantly higher average closeness centrality than insects, whereas their betweenness centrality was lower than that of insects. This is because a few insects, mainly in the bird-dominated module ( Supplementary Note 2 , Supplementary Tables 8 and 9 ), had high betweenness values as they connected the six insect-dominated modules with the bird–flower module. This latter module included most plants (58%) and 16 of the 19 birds, thus dominating the pollination network. However, a study of the pollen loads on insects would bring the insect- and bird-dominated modules closer together. We are confident to conclude that the small bird community compared with the large insect community plays a relatively important role to the pollination of the Galápagos plant community. The high network generalization level facilitates the integration of alien plants into the Galápagos bird–flower network, as has also been found in other mutualistic networks [11] , [36] . Galápagos birds included alien and native plants to the same levels into their diet and may thus enhance plant invasions on this increasingly human-altered archipelago. The enhancement of plant invasion by birds will obviously be higher in those species that depend on animal pollination for reproduction, and probably lower in those that are self- or wind-pollinated, such as P. guajava . In turn, this alien invasive species is likely to take over and disrupt interactions between birds and native plants, with unknown ecological and evolutionary consequences [37] . In fact, 56% of the samples included pollen of this species together with native pollen. Moreover, an average of 52% (s.d.=34%) of the pollen grains found on those samples were from P. guajava , suggesting heterospecific pollen interference in ovule fertilization by deposition of alien pollen on the stigmas of native plants. Pollination interactions had a high turnover across islands, which is also observed in other archipelagos, for example, the Canary Islands [38] . Causes of the high turnover include sampling incompleteness, non-overlapping geographical ranges of species, rareness, phenological mismatches, strong inter-island variation in vegetation composition and specific diet preferences across islands. Quantitative networks showed a very similar structure across Santa Cruz and San Cristóbal, lowland and highland, and hot and cold seasons ( Supplementary Fig. 3 , Supplementary Table 4 ). Thus, Galápagos birds are very opportunistic in their flower choice and search for food. The variation we did observe among islands, habitats and seasons is probably driven by differences in floral resource abundance, and consequently natural selection on bird traits might vary in a similar manner as demonstrated for the interaction between finches and their seed sources [39] . This dynamics in community interaction structure and its evolutionary potential may become an important step in our increasing understanding and appreciation of the biodiversity puzzle of the Galápagos Islands. Even though nobody has quantified arthropod biomass on the Galápagos, we share the impression of Darwin and many later naturalists, that these islands indeed are ‘so poor a country’ [1] , [40] . Thus, to survive, birds widen their niche and include other food sources, such as nectar and pollen, substantiating an interaction release. This scenario is supported by two conclusions from our study: (1) all Galápagos land birds converged in their feeding niche to visit flowers and transport their pollen, and (2) connectance was considerably higher than expected for networks of this size. The first conclusion is an astonishing finding, never reported before for any ecosystem: a massive response of the bird community towards an underexploited resource. The possibility that birds primarily visited flowers to consume insects is unlikely, as the importance of flowering plant species to birds (measured as no. of bird visits) was uncorrelated with the importance of flowering plants to insects ( r s =0.14, P =0.45, no. of plant species=29; data from [11] ). In addition, only very rarely, during our long observation period of flower visitors in the archipelago (>500 h), did we observe birds capturing insects in flowers. The second conclusion emerges from the core of plant and bird species that acted as super-generalists, boosting network connectance and repressing any tendency towards modularity. This result is of general importance to island biology and ecosystem stability [41] . Finally, we anticipate that interaction release is a widespread island phenomenon, particularly in isolated oceanic islands with simple ecological networks and disharmonic faunas. Study sites The Galápagos archipelago comprises 18 islands >1 km 2 and numerous islets. Our study focused on the 12 largest islands (excluding Baltra, ∼ 350 m off Santa Cruz; Supplementary Fig. 1 ), covering the whole spectra of age, area, elevation and level of disturbance. The arid zone in the lowlands comprises ∼ 80% of the total land cover. The flora consists of 557 native vascular species (32% endemic), and an additional 825 ( ∼ 60%) aliens [42] . The archipelago has a hot/wet season (January–May) and a cold/dry season (June–December). Observation of flower visitors We collected data during the flowering peak (February–March) from 2010 to 2013 in all 12 islands. During three consecutive days on each island we recorded bird visitation at all flowering species in an area of about 1 km 2 (see details in ref. 11 ). Overall, this effort resulted in ∼ 500 h of flower-visitor observations. Pollen transport by birds We evaluated pollen transport on mist-netted birds in the arid zone of all islands during the flowering peak, and further sampled more intensively in Santa Cruz and San Cristóbal during 2 months of each season in the two main habitats (arid, in the lowlands and humid in the highlands). Mist nets were open from sunrise until mid afternoon under favourable weather conditions, and regularly inspected for captured birds; nets operated for ∼ 600 h. Birds were individually sampled for pollen load by swabbing a small cube ( ∼ 3 mm 3 ) of glycerine jelly, stained with fuchsine, on their beak and peri-mandibular feathers (that is, throat and forehead). The gelatine cube was then placed on a microscope slide, which was covered and melted by a weak heat source to produce a single layer of stained pollen grains. Preparations ( n =769) were sealed with clear nail polish, labelled and stored. Pollen grains were later identified by means of a reference collection and counted under a light contrast Zeiss microscope. Interaction networks The qualitative ‘archipelago network’ included direct and indirect evidence of bird–flower visits from the 12 study islands. Four network metrics were obtained to describe its topology: linkage level, connectance, nestedness and modularity ( Supplementary Note 1 ). For the more intensively sampled networks, Santa Cruz and San Cristóbal, we built quantitative matrices in which interaction weight was the number of samples in which pollen of any given plant species were identified (that is, frequency of occurrence). For these quantitative networks, we calculated the above parameters and, in addition, specialization level d ′, species strength, interaction evenness, weighted nestedness WNODF and H 2 ′. Except for nestedness and modularity, all metrics were obtained using the R package bipartite v. 2.01 (refs 43 , 44 ). General linear models were used to compare the species-level network metrics between islands, habitats, seasons, plant origin and bird functional group. For the last comparison, we included bird abundance as a covariate in the models. Evaluation of sampling completeness of interactions We aimed to determine the extent to which the number of individuals sampled per bird species allowed for a sufficient description of species linkage level ( L a ). Therefore, we estimated the number of interactions accumulated as sampling effort increased separately for each bird species. We first computed sampled-based rarefaction curves for each species [45] using the package vegan (version 2.0–6) [46] in R (v. 2.15.0). Following Chacoff et al . [47] , for each of the 13 bird species from which we had obtained a minimum of 10 samples, we calculated the percentage of estimated asymptotic richness detected as, % S OBS =100* S OBS / S E , where S OBS is the observed pollen richness in the samples (that is, birds’ linkage level, L a ) and S E is the asymptotic estimated pollen richness (that is, estimated bird L a ). To compute S E , we used the Chao 2 non-parametric estimator, S E = S OBS +[ L 2 /2 M ], where L is the number of species that occur in only one sample (‘unique’ species), M is the number of species that occur in exactly two samples and S OBS is the observed number of species [48] . Chao 2 index relies on the principle that rare species in the samples carry most information on the number of un-observed species [49] and it is one of the more robust estimators for small sample sizes [50] . How to cite this article: Traveset, A. et al . Bird–flower visitation networks in the Galápagos unveil a widespread interaction release. Nat. Commun . 6:6376 doi: 10.1038/ncomms7376 (2015).